Large fibre size in skeletal muscle is metabolically advantageous Skeletal muscle fibre size is highly variable, and while diffusion appears to limit maximal fibre size, there is no paradigm for the control of minimal size. The optimal fibre size hypothesis posits that the reduced surface area to volume in larger fibres reduces the metabolic cost of maintaining the membrane potential, and so fibres attain an optimal size that minimizes metabolic cost while avoiding diffusion limitation. Here we examine changes during hypertrophic fibre growth in metabolic cost and activity of the Na + -K + -ATPase in white skeletal muscle from crustaceans and fishes. We provide evidence for a major tenet of the optimal fibre size hypothesis by demonstrating that larger fibres are metabolically cheaper to maintain, and the cost of maintaining the membrane potential is proportional to fibre surface area to volume. The influence of surface area to volume on metabolic cost is apparent during growth in 16 species spanning a 20-fold range in fibre size, suggesting that this principle may apply widely. Although it is generally accepted that cell size is regulated, the mechanisms that govern cell size are poorly understood [1] , [2] , [3] . Skeletal muscle fibres are multi-nucleated syncytia that are among the largest cell types, and across the animal kingdom range in diameter from several microns to thousands of microns. The maximal fibre size seems to be limited by diffusion constraints associated with aerobic metabolism, which relies on the transport of O 2 from the blood to the mitochondria and subsequent diffusion of ATP from mitochondria to cellular ATPases [3] , [4] , [5] . In contrast, there is no paradigm to explain the limitations on minimal fibre size. This is a substantial gap in understanding, as many skeletal muscle fibre types attain sizes that make them nearly diffusion limited, suggesting that they may be under selective pressure to be as large as possible [4] , [5] . For instance, some skeletal muscle fibres undergo structural changes during hypertrophic increases in fibre size, such as mitochondrial and nuclear redistribution or shifts in growth patterns [4] , [5] , [6] , [7] , [8] , [9] , and reaction-diffusion models have demonstrated that these changes are necessary to offset the increasing diffusion constraints associated with fiber growth [6] , [7] , [10] , [11] , [12] . Thus, there are structural and metabolic responses that allow fibres to grow larger than would otherwise be possible while still retaining full function. In an effort to explain the very large fibres found in white muscle of some cold-water fishes, Johnston et al . [13] , [14] , [15] proposed the ‘optimal fibre size hypothesis’, which states that fibre size represents a balance between the need for small fibres that promote rapid diffusive flux and potential metabolic cost savings associated with large fibres that have a low surface area to volume (SA:V) over which to maintain the membrane potential. Muscle represents a large fraction of body mass in many animals, and in humans accounts for 20–30% of total resting O 2 consumption [16] . A major source of ATP demand in muscle is maintenance of the membrane potential by the Na + -K + -ATPase [17] , and this is the only sizable ATP sink in resting muscle that is associated with the sarcolemmal membrane and therefore potentially sensitive to fibre SA:V. We previously found that in lobster abdominal muscle that undergoes hypertrophic fibre growth, the smaller fibres of juvenile animals had a two-fold higher SA:V than the much larger fibres of adults, and this was associated with a two-fold higher ATP cost of the Na + -K + -ATPase (in resting muscle preparations) and a two-fold higher maximal enzyme activity of the Na + -K + -ATPase (in muscle homogenates) [18] . These results suggested that the very large fibres found in this species are advantageous because of a reduced SA:V, as proposed by Johnston et al . [13] , [14] , [15] However, it remains unclear whether this is a general principle that applies over a broad fibre size range. The present study tested whether larger fibres are cheaper to maintain by evaluating the fibre SA:V-dependence of Na + -K + -ATPase cost and maximal activity in white muscle from small and large size classes of 16 species of crustaceans and fishes. White muscle from these groups was selected because it typically grows hypertrophically in crustaceans [4] , [8] , [19] and fishes [5] , [20] , [21] , constitutes a large fraction of body mass, and is used relatively infrequently for burst contraction. Therefore, economy of maintenance of resting muscle may be under particularly strong positive selection in these groups. Further, in some species hypertrophic growth is coupled to a very large increase in post-metamorphic body mass, leading to dramatic increases in fibre size during animal growth. By examining changes in Na + -K + -ATPase cost and activity during growth within species, we were able to account for variation linked to phylogeny. The 16 species selected had a large range in mean body mass and mean fibre size both within and between species, and included a phylogenetically diverse group of marine and freshwater animals, allowing us to test the hypothesis that large fibres are cheaper to maintain. The absolute and fractional ATP cost in resting muscle, and the maximal enzyme activity of the Na + -K + -ATPase in muscle homogenates were proportional to changes in SA:V, providing the first experimental evidence across a wide range of fibre sizes and species that large fibre size is likely metabolically advantageous. This may explain why many fibres grow to sizes that put them on the brink of diffusion limitation. 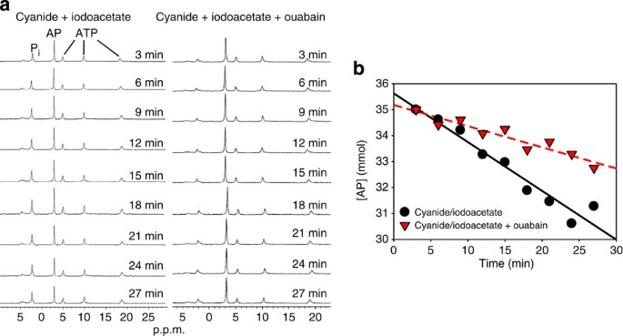Figure 1: Example of31P-NMR measurement of AP depletion rates. Representative experiment showing changes over time in (a) NMR spectra and (b) AP concentration during treatment with CN and IA or CN, IA and OU. The AP depletion rate was higher when energy metabolism alone was blocked with CN and IA than when energy metabolism and the Na+-K+-ATPase were inhibited with CN, IA and OU. The CN and IA treatment yields the total ATP demand, and the difference between slopes is the ATP cost of the Na+-K+-ATPase in isolated resting muscle. Body mass and fibre size The species examined, body masses and fibre sizes for each size class are shown in Table 1 . In each species, there was no overlap in the body mass range of the small and large size classes, but there was some overlap in fibre diameter range between size classes primarily due to the presence of some small fibres in each large size class. Across species, the mean body mass ranged from <0.1 g to 687 g (a nearly 7,000-fold range) and mean fibre size ranged from 38 to 763 μm (a 20-fold range). As SA:V of a cylinder (excluding the ends) is 2/radius, this corresponds to a 20-fold range in fibre SA:V. For both body mass and fibre size there was a significant effect of species ( P <0.0001 for both, Kruskal–Wallis tests) and size class when all species were pooled ( P <0.0001 for both, Wilcoxon tests). Pairwise comparisons indicated that body mass and white muscle fibre diameter from every species was significantly greater in the large size class than in the small size class (Wilcoxon tests with significance level adjusted for multiple comparisons; see Methods ), indicative of hypertrophic fibre growth ( Table 1 ). Table 1 Species and size class information. Full size table ATP cost and maximal activity of the Na + -K + -ATPase To calculate the ATP cost of the Na + -K + -ATPase in resting muscle, the rate of depletion of phosphocreatine (PCr; fishes) or arginine phosphate (AP; crustaceans) was measured in small muscle preparations using 31 P-NMR. 31 P-NMR spectra were collected while energy metabolism was inhibited with cyanide (CN) and iodoacetate (IA), and the rate of PCr or AP depletion was used to determine the total ATP demand in the resting muscle. Here, the rate of PCr or AP consumption is equivalent to the rate of resting ATP demand. These experiments were repeated under identical conditions (CN and IA were again used to inhibit energy metabolism), except that ouabain (OU) was also added to inhibit the Na + -K + -ATPase. The reduction in the PCr or AP depletion rate when OU was added was used to calculate the absolute Na + -K + -ATPase energetic cost (mM of ATP hydrolysed per min) as well as the fraction of total ATP consumption attributable to the Na + -K + -ATPase in isolated resting muscle (see Methods ). In separate experiments, the maximal enzyme activity of the Na + -K + -ATPase was measured in muscle homogenates to determine whether the total capacity for Na + and K + transport was also dependent on fibre SA:V (see Methods ). The small muscle preparations displayed good metabolic stability during NMR experiments, based on high initial PCr or AP to ATP ratios, and low inorganic phosphate (P i ) in the spectra from all species ( Fig. 1a ). In some representative species ( P. argus , H. americanus , C. sapidus and C. striata ), additional experiments were run where tissues were maintained in oxygenated saline to ensure that there was no change in PCr or AP concentration over the 30 min time course of the NMR experiments. In contrast, addition of inhibitors of oxidative phosphorylation (CN) and glycolysis (IA) produced linear reductions in PCr or AP over time (and corresponding increases in P i ), and when OU was simultaneously added the rate of PCr or AP depletion was reduced ( Fig. 1b ), allowing us to determine the absolute and fractional cost of the Na + -K + -ATPase in resting muscle from the difference in the slopes. Figure 1: Example of 31 P-NMR measurement of AP depletion rates. Representative experiment showing changes over time in ( a ) NMR spectra and ( b ) AP concentration during treatment with CN and IA or CN, IA and OU. The AP depletion rate was higher when energy metabolism alone was blocked with CN and IA than when energy metabolism and the Na + -K + -ATPase were inhibited with CN, IA and OU. The CN and IA treatment yields the total ATP demand, and the difference between slopes is the ATP cost of the Na + -K + -ATPase in isolated resting muscle. 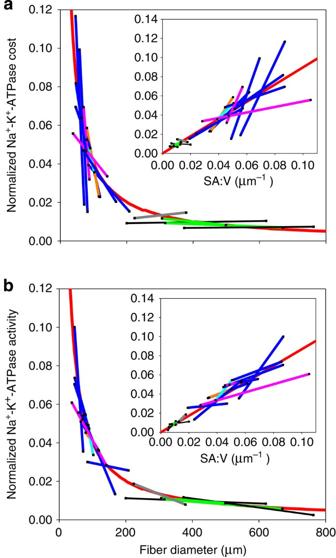Figure 2: Na+-K+ATPase cost and enzymatic activity during hypertrophic fibre growth. (a) Absolute Na+-K+ATPase cost and (b) maximal enzymatic activity, normalized to fit all species on a single plot. The straight coloured lines connect the mean values for the small and large size classes (for visualization purposes only) and show that the changes in cost and activity during hypertrophic growth follow the pattern predicted for SA:V (red line) over a wide fibre size range. The data were normalized by dividing the absolute cost of the Na+-K+ATPase (Table 2) by the adjustable coefficient, α, the value of which was determined for each species from an iterative curve fit as described inSupplementary Fig. S1, allowing all data to be plotted in a single graph. The line colour represents species group (pink=marine shrimp, green=marine lobster, grey=freshwater crayfish, black=marine crab, blue=marine teleost fish, cyan=freshwater teleost fish and orange=marine elasmobranch). The insets are the same data plotted as a linear function of SA:V (linear regression equations: normalized cost=0.942(SA:V)+0.002,r2=0.72,P<0.0001 (t-test,n=32); normalized activity=0.812(SA:V)+0.003,r2=0.86,P<0.0001 (t-test,n=32)). Full size image Table 2 presents the PCr and AP mean depletion rates and calculated absolute and fractional costs of the Na + -K + -ATPase in resting muscle, along with the Na + -K + -ATPase maximal activity in muscle homogenates. Kruskal–Wallis analyses revealed the effects of species on PCr and AP depletion rate in both size classes (small: P =0.0084; large: P <0.0001), and Wilcoxon tests found significant differences between inhibitor treatments in both size classes (small: P <0.0001; large: P <0.0001). The species effect is largely related to the much higher depletion rates in crustaceans than in fishes. The difference between treatments reflects the fact that the mean depletion rate was lower when OU was added in every species and size class, as expected, although pairwise comparisons within species were not significant following adjustment of the significance level for multiple tests. The absolute and fractional Na + -K + -ATPase cost is derived from differences in the mean depletion rates, and therefore has no error, but in 13 of 16 species (absolute) and 14 of 16 species (fractional) the Na + -K + -ATPase cost was lower in the large size class. When these data were pooled across species, the absolute cost ( P =0.035) and fractional cost ( P =0.019) were significantly lower in the large size class as expected (Wilcoxon tests). The Na + -K + -ATPase activity in muscle homogenates had a similar pattern, where a significant effect of species was found ( P <0.0001; Kruskal–Wallis test), and there was a significant difference between size classes when all of the species were pooled ( P <0.0001; Wilcoxon test). In every species, the large size class had lower activity, which accounts for the size class difference, although pairwise comparisons revealed that most of these differences within a species were not significant following adjustment of the significance level for multiple tests (Wilcoxon tests, Table 2 ). Table 2 PCr or AP depletion rates and Na + -K + -ATPase cost and maximal activity. Full size table Na + -K + -ATPase cost and activity are dependent on SA:V Supplementary Figure S1 shows the mean fibre sizes and mean fractional cost and activity measurements for the small and large size class of each species fitted to a SA:V curve (data from Tables 1 and 2 ). As hypothesized, the changes in Na + -K + -ATPase fractional cost in resting muscle ( Supplementary Fig. S1a ) and activity in homogenates ( Supplementary Fig. S1b ) during hypertrophic fibre growth were proportional to changes in SA:V. The same pattern exists for absolute Na + -K + -ATPase cost, and when these data were normalized to show all species on a single plot, it is clear that the absolute ATP cost ( Fig. 2a ) and enzyme activity ( Fig. 2b ) demonstrate SA:V dependence over a broad fibre size range. There clearly is some deviation from the SA:V dependence, which likely arises from experimental and biological variation. However, the fact that fundamentally different types of measurements of fractional/absolute cost ( Fig. 2a and Supplementary Fig. S1a ) in intact resting muscle and maximal activity in homogenates ( Fig. 2b and Supplementary Fig. S1b ) yield the same pattern provides strong support for our methodology and conclusions that larger fibres are cheaper to maintain. Figure 2: Na + -K + ATPase cost and enzymatic activity during hypertrophic fibre growth. ( a ) Absolute Na + -K + ATPase cost and ( b ) maximal enzymatic activity, normalized to fit all species on a single plot. The straight coloured lines connect the mean values for the small and large size classes (for visualization purposes only) and show that the changes in cost and activity during hypertrophic growth follow the pattern predicted for SA:V (red line) over a wide fibre size range. The data were normalized by dividing the absolute cost of the Na + -K + ATPase ( Table 2 ) by the adjustable coefficient, α, the value of which was determined for each species from an iterative curve fit as described in Supplementary Fig. S1 , allowing all data to be plotted in a single graph. The line colour represents species group (pink=marine shrimp, green=marine lobster, grey=freshwater crayfish, black=marine crab, blue=marine teleost fish, cyan=freshwater teleost fish and orange=marine elasmobranch). The insets are the same data plotted as a linear function of SA:V (linear regression equations: normalized cost=0.942(SA:V)+0.002, r 2 =0.72, P <0.0001 ( t -test, n =32); normalized activity=0.812(SA:V)+0.003, r 2 =0.86, P <0.0001 ( t -test, n =32)). Full size image The present study provides experimental evidence in a broad range of species and fibre sizes that large fibres are metabolically advantageous because they are cheaper to maintain. The reduced maintenance costs of larger fibres may also explain prior findings that indicate that many fibres are on the brink of diffusion limitation in adult animals (reviewed in Kinsey et al . [5] ). During hypertrophic fibre growth in white muscle of fishes and crustaceans, there is a dramatic shift in the distribution of mitochondria from the fibre interior to the periphery, which limits O 2 diffusion distances and enhances aerobic metabolic rates, and an opposing shift in nuclei from the fibre periphery to the interior, which limits macromolecular diffusion distances within the myonuclear domain and enhances rates of protein turnover [4] , [5] , [6] , [7] , [8] , [9] , [10] , [11] , [12] . Thus, these organelle distribution shifts during fibre growth allow the fibres to grow larger than would otherwise be possible. Modelling indicated that aerobic metabolism is the most important limiter of fibre size, and that if fibres were to continue to grow hypertrophically beyond the maximal size found in adults, aerobic metabolism would become substantially diffusion limited. In fact, in white muscle from black sea bass ( Centropristis striata ), as the animal grows to near maximal body size and our models predict that further fibre growth would result in diffusion limitation, the muscle fibres shift from exclusively hypertrophic growth to largely hyperplasic growth and/or fibre splitting [9] . These and other prior results, when coupled with the findings of the present study, are consistent with the optimal fibre size hypothesis, where fibres reach a maximal size that minimizes maintenance cost without becoming constrained by diffusion. Johnston et al . [13] , [14] , [15] originally proposed the optimal fibre size hypothesis to explain the presence of very large white fibres in some cold-water fishes, but the influence of fibre size on SA:V is actually greatest in small fibres. Fibres with a maximal diameter less than about 100 μm had a large decrease in both cost and activity during hypertrophic growth, while the absolute cost savings associated with continued growth to hundreds of microns is smaller ( Fig. 2 ). Thus, the metabolic advantages of hypertrophic fibre growth are likely greatest in animals with relatively small fibres, including mammals and birds, where the typical increase in fibre size during animal growth would lead to a large change in SA:V. Further, most muscles grow by a combination of hyperplasia and hypertrophy, and the linkage between muscle growth pattern and metabolic rate suggests that the activation of hyperplasic growth that produces small fibres would also lead to an elevation of muscle, and likely whole animal, resting metabolic rate. The present study provides evidence for a key component of the optimal fibre size hypothesis, but does not demonstrate that maximizing fibre size is under positive selective pressure as proposed previously [13] , [14] , [15] . However, prior work has shown that diversity in body size attained following post-glacial invasions of freshwater habitats by fishes was associated with parallel changes in muscle growth patterns in a manner consistent with a shift toward a more optimal fibre size [22] . In Arctic charr and threespine stickleback selection for dwarfism is associated with a dramatic reduction in the maximal number of fibres in muscle (by as much as 85% in Arctic charr). That is, as the maximal adult body mass is reduced fewer fibres are needed to meet the demands for muscle growth. This leads to an adult fibre diameter that is greatly increased in the dwarf populations over what it would have been had there not been a reduction in new fibre formation. In Arctic charr, the adaptive increase in adult fibre size of the dwarf population reduced the SA:V by up to 35%, which would be expected to reduce the cost of maintaining ionic gradients across the sarcolemma by a similar amount. In a rapidly evolving population of dwarf sticklebacks, adaptation of new fibre recruitment patterns occurred within ~10 generations, suggesting that there is intense selection for optimal fibre size in this population [22] . Similarly, the very large fibre size among many members of the notothenioid lineage of fishes appears to be a mechanism to reduce energy demand and is associated with adaptation to the cold water of the Southern Ocean. In this case, the very low metabolic demands of the muscle tissues relax diffusion constraints, allowing the fibres to grow to extreme dimensions [13] . Although the data were normalized in Fig. 2 so that all species could be plotted on a single SA:V curve, there was a strong phylogenetic signature in all of the results ( Table 2 ). This was most obvious when comparing the two major groups of animals, where Na + -K + -ATPase absolute cost, fractional cost and activity, as well as the total ATP demand in resting muscle (the IA+CN treatments in Table 2 ), were higher in muscle from crustaceans than fishes (Wilcoxon tests, P <0.0006 for all). For example, in crustaceans the Na + -K + -ATPase cost accounted for an average of 57±3% of the total energy expenditure in resting muscle from the small size classes of animals, and 45±4% of total energy expenditure in the large size classes. In fishes, the Na + -K + -ATPase accounted for 35±4% of the total ATP demand in resting muscle from animals in the small size classes, but only 15±3% in the large size classes. The greater effect of hypertrophic growth on ATP cost seen in the fishes compared with crustaceans reflects the fact that the fish species examined generally had smaller fibres than the crustaceans, so small increases in fibre size led to large changes in SA:V. The fractional costs of the Na + -K + -ATPase measured in the present study were consistent with previous results from studies in skeletal muscle from sheep [23] , calves [23] , mice [24] , rats [25] and lugworms [26] . Thus, the Na + -K + -ATPase cost represented a sizable fraction of the total resting ATP demand, indicating that reducing fibre SA:V can lead to a substantial energetic saving. The phylogenetic dependence of the data illustrate the importance of examining the change in cost and activity associated with fibre growth within each species, as the SA:V dependence is otherwise not apparent. Although there was considerable variation among species the absolute Na + -K + -ATPase cost was linearly dependent on the maximal activity across all species and size classes (cost=0.0028 × activity+0.025, r 2 =0.25, P =0.0038; data in Table 2 ). This is consistent with the linear dependence of skeletal muscle oxygen consumption on Na + -K + -ATPase activity in rat [25] . The implication of this finding is that the number of Na + -K + -ATPase pumps largely dictates cost, and within a species pump density does not change during growth and total pump number parallels total sarcolemmal surface area ( Fig. 2 and Supplementary Fig. S1 ). Therefore, reducing the expression of the Na + -K + -ATPase does not appear to be a strategy to reduce costs in the smaller fibres of the small size class animals. In summary, this study provides the first direct evidence over a broad range of species and fibre sizes that large fibres are advantageous because they are cheaper to maintain. These results, coupled with prior work indicating that large fibre size is under positive selection and that fibres often attain a maximal size that is on the brink of diffusion limitation, are consistent with the optimal fibre size hypothesis proposed by Johnston et al . [13] , [14] , [15] The present study also suggests that there is a link between fibre size and whole animal metabolic rate. Animal collection and fibre diameter measurements Small and large size classes of fishes and crustaceans were collected locally or supplied by vendors. Fibre diameter and body mass of each species and size class were measured according to previous protocols from Hardy et al . [7] and Jimenez et al . [10] , [18] All procedures were approved by the University of North Carolina Wilmington Institutional Animal Care and Use Committee. Total ATP demand and Na + -K + -ATPase cost in resting muscle The total resting ATP demand and the demand of the Na + -K + -ATPase were determined in small isolated preparations, ~1 mm in diameter, of anterior epaxial muscle in fishes [6] , abdominal extensor muscle in shrimp, lobsters and crayfish [10] , [18] and fifth periopod light levator muscle from crabs [7] , [8] . The muscle preparations were secured at resting length to the outside of a section of rigid superperfusion tubing (1 mm OD) and saline flow was provided by peristaltic pumps. The rigid section of tubing with the muscles attached was inserted into a 5-mm NMR tube so that flow through the superfusion tubing entered at the bottom of the NMR tube and exited via a separate superfusion tube at the top, thus washing over the muscle preparation [18] . The rate of decrease of PCr or AP was monitored over time with 31 P-NMR in the presence of metabolic inhibitors [18] . PCr and AP are substrates in the creatine kinase (CK) and arginine kinase (AK) reactions, respectively, which catalyse the transfer of a phosphoryl group from PCr or AP to ADP, forming ATP. CK and AK have high activity that far exceeds the ATP turnover rate in resting white muscle, so the substrates and products of the reactions are maintained at equilibrium, and there is a 1:1 stoichiometry of PCr hydrolysed to ATP formed. Therefore, if ATP supply is inhibited, PCr or AP concentration will decrease as ATP is consumed by cellular processes such as the Na + -K + -ATPase. In the present case, the total resting ATP demand was determined from the rate of PCr or AP decrease while energy metabolism was inhibited with 2.5 mM CN to block oxidative phosphorylation and 1 mM IA to block glycolysis in the appropriate saline solution [27] , [28] , [29] , [30] . The ATP cost of the Na + -K + -ATPase was determined from the reduction in the rate of PCr or AP depletion when energy metabolism was blocked as above, while simultaneously treating the muscle with 5 mM OU, which inhibits the Na + -K + -ATPase ( Fig. 1 ). A total of 339 NMR rate measurements were performed, where NMR spectra were collected every 3 min on a Bruker 400 or 600 MHz DMX spectrometer to determine relative concentrations of PCr or AP, ATP and P i . Peak areas were converted to concentration by assuming a total high-energy phoshate concentration of 50 mM. Linear regression was used to measure the rate of PCr or AP depletion. Na + -K + -ATPase maximal activity in muscle homogenates A K + -stimulated 3- O -methylfluorescein phosphatase assay was used to measure Na + -K + -ATPase maximal activity in muscle homogenates as described previously [10] , [31] , [32] , [33] . Activity was determined using spectrofluorometry at an excitation wavelength of 475 nm and an emission wavelength of 515 nm (Promega Luminometer 20/20 with a Glomax blue module; Madison, WI, USA), on small tissue sample homogenates from each size class and species. The addition of 160 μmol l –1 3- O- methylfluorescein phosphate led to a linear increase in fluorescence, which was recorded and followed by addition of 10 μmol l –1 KCl to activate the Na + -K + -ATPase. K + -dependent 3- O -methylfluorescein phosphatase activity (that is, Na + -K + -ATPase activity) was determined by subtracting activity before the addition of KCl from activity after the addition of KCl. Statistical analyses Data were non-normally distributed and could not be transformed to meet this assumption so all analyses were conducted using non-parametric tests. For body mass, fibre size and Na + -K + -ATPase activity, Kruskal–Wallis analyses were used to test for effects of species, and Wilcoxon tests were used to compare size classes when all species were pooled (overall size effect), as well as for pairwise comparisons between size classes within each species. In the latter comparisons, we adjusted the significance level to account for multiple tests of the same hypothesis following the procedures of Hochberg [34] . To evaluate the PCr and AP depletion rate data, Kruskal–Wallis tests were used to test for significant effects of species within each size class, and Wilcoxon tests were used to test for differences between treatments (CN+IA or CN+IA+OU) within each size class when all species were pooled. Pairwise comparisons were made to test for differences between treatments (CN+IA or CN+IA+OU) within each species and size class using Wilcoxon tests, again adjusting for multiple tests. The Na + -K + -ATPase absolute cost and fractional cost were derived from mean PCr or AP depletion rates and therefore had no error term, preventing a comparison of size classes within species. However, Wilcoxon tests were used to compare the size classes when the absolute and fractional cost data were pooled across species. Results were considered significant if P <0.05, except in cases where significance levels were adjusted as described above [34] . How to cite this article: Jimenez, A.G. et al . Large fibre size in skeletal muscle is metabolically advantageous. Nat. Commun. 4:2150 doi: 10.1038/ncomms3150 (2013).